Chronic lung diseases are associated with gene expression programs favoring SARS-CoV-2 entry and severity Patients with chronic lung disease (CLD) have an increased risk for severe coronavirus disease-19 (COVID-19) and poor outcomes. Here, we analyze the transcriptomes of 611,398 single cells isolated from healthy and CLD lungs to identify molecular characteristics of lung cells that may account for worse COVID-19 outcomes in patients with chronic lung diseases. We observe a similar cellular distribution and relative expression of SARS-CoV-2 entry factors in control and CLD lungs. CLD AT2 cells express higher levels of genes linked directly to the efficiency of viral replication and the innate immune response. Additionally, we identify basal differences in inflammatory gene expression programs that highlight how CLD alters the inflammatory microenvironment encountered upon viral exposure to the peripheral lung. Our study indicates that CLD is accompanied by changes in cell-type-specific gene expression programs that prime the lung epithelium for and influence the innate and adaptive immune responses to SARS-CoV-2 infection. In December 2019, a respiratory disease associated with a novel coronavirus emerged in Wuhan, China [1] , [2] , [3] . The syndrome, now called COVID-19, was caused by severe acute respiratory syndrome coronavirus 2 (SARS-CoV-2) and has since rapidly spread worldwide [4] . As of May 18, 2021, a total of over 163 million confirmed COVID-19 cases and more than 3.3 million deaths have been reported around the globe [5] . The clinical manifestations of SARS-CoV-2 infection range from asymptomatic to fulminant cases of acute respiratory distress syndrome (ARDS) and life-threatening multi-system organ failure. Development of ARDS in patients with SARS-CoV-2 dramatically increases the risk of ICU admission and death [6] , [7] , [8] , [9] , [10] , [11] , [12] . Risk factors for severe SARS-CoV-2 include age, smoking status, ethnicity and male sex [13] , [14] , [15] . Baseline comorbidities including hypertension, diabetes and obesity, increase SARS-CoV-2 susceptibility and severity [1] , [10] , [16] , [17] , [18] , [19] . In addition, chronic lung disease (CLD) has been identified as a risk factor for hospitalization and mortality in patients with COVID-19 [20] , [21] , [22] , [23] , [24] , [25] , [26] , [27] . Patients with chronic obstructive pulmonary disease (COPD) and interstitial lung disease (ILDs), especially Idiopathic Pulmonary Fibrosis (IPF), have a significantly higher COVID-19 mortality rate compared to patients without chronic lung disease [28] . However, the molecular mechanisms underlying the increased risk of SARS-CoV-2 severity and mortality in patients with pre-existing lung diseases are not well understood. In this work, we performed an integrated analysis of four lung single cell RNA-sequencing (scRNA-seq) datasets [29] , [30] , [31] , [32] in addition to unpublished data, together including 78 control and 132 CLD samples ( n = 31 COPD, 82 IPF and 19 other ILDs), to investigate the molecular basis of SARS-CoV-2 severity and mortality risk in CLD patients. We found that CLD is associated with baseline changes in cell-type specific expression of genes related to viral replication and the immune response, as well as evidence of immune exhaustion and altered inflammatory gene expression. Together, these data provide a molecular framework underlying the increased risk of SARS-CoV-2 severity and poor outcomes in patients with certain pre-existing CLD. 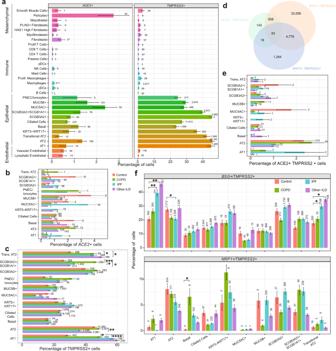Fig. 1: Percentage of cells expressing SARS-CoV-2 receptor genes in lung cell types in different diagnosis subgroups. aPercentage of cells expressingACE2andTMPRSS2in all cell types. Numbers are the total number ofACE2+ orTMPRSS2+ cells in each cell type in the dataset.b,cPercentage of cells expressingACE2(b) andTMPRSS2(c) in each diagnosis group in the epithelial cell types.dVenn diagram shows overlapping of cells co-expressing the proposed receptors (ACE2,BSGandNRP1) and the proteaseTMPRSS2.e,fPercentage of cells co-expressing receptors andTMPRSS2split by cell type and diagnosis group. Plots were generated with mean values of percentage of cells per individual samples, and data are presented as mean values ± SEM. Significant differences between diagnosis groups were calculated using Tukey_HSD test,pvalue < 0.05: *pvalue < 0.01: **pvalue < 0.001: ***pvalue < 0.0001: ****. Integrated analysis of lung single cell RNA sequencing datasets To determine why COVID-19 patients with CLD have a higher risk of severe infection and poorer outcomes, we performed an integrated analysis on four published scRNA-seq lung datasets: Northwestern (biopsy deemed representative of explanted lung), Pittsburgh and VUMC/TGen (biopsy of apical and basal region of explanted lung) and Yale/BWH (longitudinal biopsy through explanted lung) (Supplementary Table 1a ), in addition to previously unpublished samples (VUMC/TGen). We analyzed the transcriptomes from 611,398 single cells derived from healthy donors (78 samples), COPD (31 samples), IPF (82 samples) and Non-IPF ILD (Other ILD, 19 samples) (Supplementary Table 1b , 2 ). 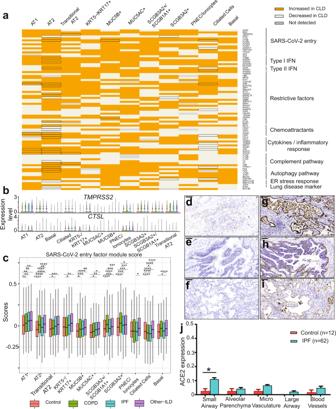Fig. 2: Expression profile of SARS-CoV-2 mediators and response genes in the epithelial cell population. aBinary heatmap representing a manually curated list of genes associated with SARS-CoV-2. Orange elements indicate genes with increased expression and white elements indicate genes with decreased expression in CLD samples; Not detected: gene expression was not detected in either of the two tested populations (CLD vs. Control). Differential expressed genes (DEGs) between CLD and control samples (FDR ≤ 0.1) are outlined in black.bViolin plot depicts gene expression level in CLD and control of the two SARS-CoV-2 proteasesTMPRSS2andCTSL.cSARS-CoV-2 entry module score in different cell types, SARS-CoV-2 mediators includedACE2, BSG (CD147), NPR1, HSPA5 (GRP78), TMPRSS2, CTSL, ADAM17, FURIN. The outliers were removed in this plot, please see Supplementary Fig.8awith outliers included. Boxes: interquartile range, lower and upper hinges correspond to the first and third quantiles, upper and lower whisker extends from the hinge to the largest values or smallest values of 1.5 x interquartile range; *pvalue < 0.05, **pvalue < 0.01, ***pvalue < 0.001, ****p-value < 0.0001, Tukey_HSD post-hoc test. ACE2 and ITGB6 protein expression in IPF lung sections. IPF lung sections stained for ACE2:dsmall airway,elarge airway andflung parenchyma. IPF lung sections stained for αvβ6:gsmall airway,hlarge airway andilung parenchyma.jSemi-quantitative evaluation of ACE2 scoring among control (n= 12 for each tissue) and IPF (n= 62 for each tissue) sections (both the percentage of staining and staining intensity of ACE2 expression; 0-Negative; 1–0–⩽10%; 2-11–⩽25%; 3-⩽26%), data are presented as mean values ± SEM. Significant differences between IPF and control were calculated using Tukey HSD test,pvalue < 0.05 *. Scale bar = 100 µm. Ford–j: a total of 12 normal lung samples and 62 IPF samples were used. Using published cell type specific markers [31] , [32] , we identified 32 distinct cell types in the dataset (Supplementary Fig. 1 ). 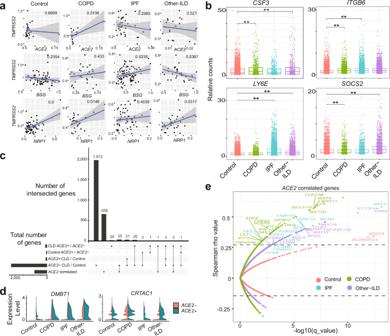Fig. 3: CLD AT2 cells exhibit baseline differences in gene expression profile coping with viral infection. aSignificant gene expression correlation in AT2 cells betweenTMPRSS2andACE2,BSG(CD147) andNPR1in COPD and IPF samples, each dot represents the average expression level of the genes of interest per sample, pairwise gene correlation analysis was done using a fitting linear model andpvalue was calculated using Anova.bBoxplot shows differences in gene expression of selected SARS-CoV-2 response genes in the AT2 cell types among different diagnosis groups, Boxes: interquartile range, lower and upper hinges correspond to the first and third quantiles, upper and lower whisker extends from the hinge to the largest values or smallest values of 1.5 × interquartile range; **pvalue-adj ≤ 0.05 (negative binomial test, corrected for Age, Ethnicity, Smoking_status and Dataset).cUpset plot shows shared differential expression genes (DEGs) between different comparisons:ACE2−CLD vs. Control,ACE2+ CLD vs. Control, CLDACE2+ vs.ACE2-, ControlACE2+ vs.ACE2-andACE2correlated genes in the AT2 cells.dUpregulation of two genes uniquely differentially expressed in the CLDACE2+ vs.ACE2−.eSpearman gene correlation analysis identified genes correlated withACE2expression in AT2ACE2+ cells in different diagnosis groups, p-value was adjusted using Benjamini-Hochberg corrections, dashed lines indicate the 99th percentile of Spearman rho values. Overall, we observed similar cell type proportions between the different datasets and diagnosis groups (Supplementary Table 3 , Supplementary Fig. 2 ), with the exception of high AT2 cell numbers in the Northwestern dataset, as expected due to the protocol favoring isolation of AT2 and macrophages (personal communication). Despite the variation in sample collection and processing at different research institutes, the similarity in cell type composition per dataset indicated the compatibility of samples and that no major sampling bias would confound an integrated analysis. Expression profile of SARS-CoV-2 associated receptors and factors in the diseased lung SARS-CoV-2 utilizes the host ACE2 , and other putative factors such as BSG, NRP1 and HSPA5 , as entry receptors and TMPRSS2 , CTSL or FURIN as priming proteases to facilitate cellular entry [33] , [34] , [35] , [36] , [37] , [38] , [39] , [40] . Consistent with prior reports analyzing normal lung tissue [33] , [34] , [41] , ACE2 and TMPRSS2 are expressed predominantly in epithelial cell types (Fig. 1a ), while other putative SARS-CoV-2 entry receptors ( BSG , NRP1 , HSPA5 ) and priming proteases ( CTSL , FURIN ) have substantially more widespread expression in nearly all cell types (Supplementary Fig. 3 ). The total number and proportion of ACE2 + cells are highest in pericytes, type 2 alveolar cells (AT2) and secretory cells, while TMPRSS2 is widely expressed in all epithelial cell types. There were no significant differences in the proportion of ACE + cells in any cell-type in CLD versus control groups (Fig. 1b ). The proportion of TMPRSS2 + AT2 cells is decreased in IPF lungs while TMPRSS2 + AT1 and Transitional AT2 cells are higher in all CLD samples; and TMPRSS2 + SCGB3A2 +/ SCGB1A + club cells are in significantly higher numbers in COPD patients compared to controls (Fig. 1c ). The putative entry factor NRP1 is expressed in more pDCs, myofibroblasts and HAS1 high fibroblasts in CLD samples compared to control (Supplementary Fig. 3 ). Fig. 1: Percentage of cells expressing SARS-CoV-2 receptor genes in lung cell types in different diagnosis subgroups. a Percentage of cells expressing ACE2 and TMPRSS2 in all cell types. Numbers are the total number of ACE2 + or TMPRSS2 + cells in each cell type in the dataset. b , c Percentage of cells expressing ACE2 ( b ) and TMPRSS2 ( c ) in each diagnosis group in the epithelial cell types. d Venn diagram shows overlapping of cells co-expressing the proposed receptors ( ACE2 , BSG and NRP1 ) and the protease TMPRSS2 . e , f Percentage of cells co-expressing receptors and TMPRSS2 split by cell type and diagnosis group. Plots were generated with mean values of percentage of cells per individual samples, and data are presented as mean values ± SEM. Significant differences between diagnosis groups were calculated using Tukey_HSD test, p value < 0.05: * p value < 0.01: ** p value < 0.001: *** p value < 0.0001: ****. Full size image Next, we compared the number of double positive cells, i.e., cells co-expressing a receptor and priming protease, in control and CLD samples. A notable fraction of cells co-expresses all established and putative entry receptors ( ACE2 , BSG , NRP1 , HSPA5 ) and proteases ( TMPRSS2 , CTSL , FURIN ); AT2 cells comprised nearly half of all such cells (43.3%) (Fig. 1d , Supplementary Fig. 4 ). While the percentage of cells co-expressing ACE2 and priming proteases ( TMPRSS2 , CTSL , FURIN ) was similar across disease subtypes, there was a significantly higher number of cells co-expressing ACE2 and FURIN in the COPD AT2 and Transitional AT2 cells (Fig. 1e , Supplementary Fig. 4 ). We detected significant differences in the number of cells co-expressing BSG , NRP1 , HSPA5 with a priming protease in CLD samples in multiple cell types (Fig. 1f , Supplementary Fig. 4 ). To examine whether CLD patients express higher levels of SARS-CoV-2 receptors and priming proteases, we performed differential expression analysis of those genes in the CLD versus control samples. The two major SARS-CoV-2 cellular entry factors, ACE2 and TMPRSS2 , have similar expression profiles in the disease and control samples. ACE2 expression is relatively low in all cell types and there were no significant differences in ACE2 expression in CLD groups compared to control (Supplementary Fig. 5 ). The putative alternative receptor NRP1 , recently confirmed as another host entry factor for SARS-CoV-2 [35] , is slightly up-regulated in the COPD macrophages, but down-regulated in both IPF and Other-ILD macrophages (Supplementary Fig. 6 ). TMPRSS2 expression is high in AT1, AT2, Transitional AT2, PNEC/ionocytes and club cells (Fig. 2b , Supplementary Fig. 5 ) and is slightly upregulated in the AT2 COPD samples (log2FC = 0.28, q value 0.04) (Supplementary Dataset 3 ), in contrast to a recent publication demonstrating decreased TMPRSS2 expression in severe COPD [42] . Two alternative priming proteases ( CTSL and FURIN ) are expressed at low level and show no significant differences in expression between control and disease samples (Fig. 2b , Supplementary Fig. 5 ). However, the SARS-CoV-2 entry gene score (calculated on the average expression levels of all SARS-CoV-2 entry factors over a random control gene set) is significantly increased in the CLD samples in many epithelial cell types, including AT1, AT2, Basal, Club cells, and KRT5-/KRT17 + cells, an ECM-producing epithelial cell type enriched in the fibrotic lung [31] , [32] (Fig. 2c , Supplementary Fig. 8a, b ). Together, these data suggest CLD is associated with modest changes in expression of established SARS-CoV-2 entry factors, and alternative mechanisms are likely additionally responsible for observed differences in outcome severity. Fig. 2: Expression profile of SARS-CoV-2 mediators and response genes in the epithelial cell population. a Binary heatmap representing a manually curated list of genes associated with SARS-CoV-2. Orange elements indicate genes with increased expression and white elements indicate genes with decreased expression in CLD samples; Not detected: gene expression was not detected in either of the two tested populations (CLD vs. Control). Differential expressed genes (DEGs) between CLD and control samples (FDR ≤ 0.1) are outlined in black. b Violin plot depicts gene expression level in CLD and control of the two SARS-CoV-2 proteases TMPRSS2 and CTSL . c SARS-CoV-2 entry module score in different cell types, SARS-CoV-2 mediators included ACE2, BSG (CD147), NPR1, HSPA5 (GRP78), TMPRSS2, CTSL, ADAM17, FURIN . The outliers were removed in this plot, please see Supplementary Fig. 8a with outliers included. Boxes: interquartile range, lower and upper hinges correspond to the first and third quantiles, upper and lower whisker extends from the hinge to the largest values or smallest values of 1.5 x interquartile range; * p value < 0.05, ** p value < 0.01, *** p value < 0.001, ****p-value < 0.0001, Tukey_HSD post-hoc test. ACE2 and ITGB6 protein expression in IPF lung sections. IPF lung sections stained for ACE2: d small airway, e large airway and f lung parenchyma. IPF lung sections stained for αvβ6: g small airway, h large airway and i lung parenchyma. j Semi-quantitative evaluation of ACE2 scoring among control ( n = 12 for each tissue) and IPF ( n = 62 for each tissue) sections (both the percentage of staining and staining intensity of ACE2 expression; 0-Negative; 1–0– ⩽ 10%; 2-11– ⩽ 25%; 3- ⩽ 26%), data are presented as mean values ± SEM. Significant differences between IPF and control were calculated using Tukey HSD test, p value < 0.05 *. Scale bar = 100 µm. For d – j : a total of 12 normal lung samples and 62 IPF samples were used. Full size image Dysregulation of viral infection and innate immune response genes in disease epithelial cells Given the relatively modest differences in SARS-CoV-2 entry factors in epithelial cells between CLD and control lungs (Fig. 2b , Supplementary Figs. 5 , 6 ), we hypothesized that rather than greatly increased cellular susceptibility to SARS-CoV-2 infection, patients with CLD are predisposed to severe lung injury due to underlying differences in epithelial gene expression in key pathways mediating the antiviral response. Focusing on the epithelial cell population (a total of 143,114 cells), we selectively examined genes that have been demonstrated in the SARS, MERS and rapidly expanding COVID-19 literature to impact viral pathogenesis. We noted that many of these genes are significantly dysregulated (Bonferroni adjusted p-value, FDR, ≤ 0.1) in several epithelial cell types (Fig. 2a ). Included are genes thought to directly impact viral replication ( TMPRSS2, NPR1, CTSB ), interferon stimulated genes (ISGs) thought to be involved in restricting viral entry and replication ( LY6E, SPATS2L ) [43] , and key regulators of the host viral response including cytokine and inflammatory response genes (IFN type I and type II receptors, SOCS1 / 2 , CCL2, CD47 ) (Fig. 2a , Supplementary Fig. 8c, d ). In addition, the complement pathway gene C3 , an important component of the innate immune response and previously found to be elevated in SARS patients [44] , and autophagy ( FGG, FGA, PTPN11 ) genes are also significantly dysregulated in many CLD epithelial cells; these pathways are important for propagating viral infection and the host response [45] , [46] , [47] . Among the epithelial cell types, AT2 cells have the largest number of significantly dysregulated genes in CLD compared to control samples (Fig. 2a ). These data suggest that there are basal differences in the expression profiles of genes regulating viral infection and the immune response in diseased epithelial cells, in particular in AT2 cells, and that this epithelial “priming” may contribute to COVID-19 severity and poor outcomes. Elevated ACE2 protein expression level in the small airways in IPF lungs To further study the expression of the major SARS-CoV-2 entry factor ACE2 in the fibrotic lungs, we examined protein levels of ACE2 in different lung regions using the anti-ACE2 ab108252 antibody (Supplementary Fig. 9a ). In agreement with the transcript quantification above and previous immunohistology analysis [48] , we detected overall low expression level of ACE2 across all tissue types in both IPF (Fig. 2d–f ) and control lung sections (Supplementary Fig. 9b, c ). Semi-quantitative evaluation of ACE2 expression scoring showed elevated ACE2 expression in all IPF sections compared to control, reaching statistical significance in the IPF small airway sections (Fig. 2j ), suggesting that while overall ACE2 expression is low, there is a regional concentration of ACE2 + cells within the distal IPF lung that may promote a more severe localized viral response. Upregulation of the epithelial integrin alpha-V beta-6 (αvβ6) plays an important role in enhanced fibrosis in response to lung injury [49] , and enhances TGFβ activation which can suppress type I interferon responses from alveolar macrophages increasing susceptibility to viral infection [50] . We detected a significant increase of αvβ6 integrin expression in all lung sections isolated from IPF patients (Fig. 2g–i ). While there was additional positive staining in the peripheral lung, αvβ6 expression is highest in the AT2 epithelial cells in the IPF samples compared to overall low expression level in the normal lung sections (Supplementary Fig. 9b, c ), mirroring the expression data of ITGB6 described below (Fig. 3b ). Fig. 3: CLD AT2 cells exhibit baseline differences in gene expression profile coping with viral infection. a Significant gene expression correlation in AT2 cells between TMPRSS2 and ACE2 , BSG ( CD147 ) and NPR1 in COPD and IPF samples, each dot represents the average expression level of the genes of interest per sample, pairwise gene correlation analysis was done using a fitting linear model and p value was calculated using Anova. b Boxplot shows differences in gene expression of selected SARS-CoV-2 response genes in the AT2 cell types among different diagnosis groups, Boxes: interquartile range, lower and upper hinges correspond to the first and third quantiles, upper and lower whisker extends from the hinge to the largest values or smallest values of 1.5 × interquartile range; ** p value-adj ≤ 0.05 (negative binomial test, corrected for Age, Ethnicity, Smoking_status and Dataset). c Upset plot shows shared differential expression genes (DEGs) between different comparisons: ACE2− CLD vs. Control, ACE2 + CLD vs. Control, CLD ACE2 + vs. ACE2- , Control ACE2 + vs. ACE2- and ACE2 correlated genes in the AT2 cells. d Upregulation of two genes uniquely differentially expressed in the CLD ACE2 + vs. ACE2− . e Spearman gene correlation analysis identified genes correlated with ACE2 expression in AT2 ACE2 + cells in different diagnosis groups, p-value was adjusted using Benjamini-Hochberg corrections, dashed lines indicate the 99th percentile of Spearman rho values. Full size image CLD specific ACE2 + transcriptional profiles in AT2 cells In the distal lung, AT2 cells have been proposed to be the primary targets of SARS-CoV-2 [34] , [41] , [51] and comprise the initial microenvironment the virus encounters. Thus, we examined the gene expression profile of CLD AT2 cells in more detail. As described above, AT2 cells in all diagnosis subgroups have significantly higher SARS-CoV-2 entry gene scores than control cells (Fig. 2c ). In addition, CLD AT2 cells express higher levels of many genes related to viral infection and innate immune responses than any epithelial cell type (Fig. 2a ). COPD and Other-ILD, but not IPF, AT2 cells express higher levels of CSF3 , an important cytokine in the regulation of granulocytes, and the suppressor of cytokine signaling-2 ( SOCS2 ) (Fig. 3b ). The epithelial integrin ITGB6 , involved in wound healing and pathogenic fibrosis [52] , is upregulated in COPD and IPF AT2 cells; the ISG lymphocyte antigen 6 complex ( LY6E ), known to restrict SARS-CoV-2 entry [43] , [53] , is upregulated in the IPF and Other-ILD AT2 cells (Fig. 3b , Supplementary Fig. 8e ). Gene correlation analysis showed strong positive correlation between TMPRSS2 and ACE2 , NRP1 in COPD AT2 cells (Fig. 3a , Supplementary Fig. 10 ). NRP1 expression is also positively correlated with the protease FURIN in the AT2 cells isolated from IPF samples (Supplementary Fig. 10c ). Since ACE2 is the best-establishedSARS-CoV-2 entry factor, and AT2 cells accounted for 54.63% of all ACE2 + epithelial cells, we focused on the transcriptional profile of ACE2 + AT2 cells. All of the 34 differentially expressed genes (FDR ≤ 0.1) in ACE2 + AT2 cells between CLD and control overlapped with the ACE2 - cells CLD vs. control analysis (Fig. 3c ), suggesting that these genes reflected the disease state and were not related to ACE2 expression. However, when we performed the same differential expression analysis on ACE2 + vs. ACE2- CLD cells, we identified 20 unique genes that were dysregulated in CLD ACE2 + cells (Fig. 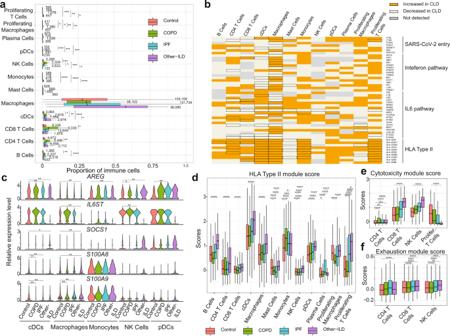Fig. 4: Analysis of SARS-CoV-2 candidate immune response genes in immune cells. aQuantification of cell types as a percent of all immune cells in control and diseased lungs, numbers represent the total numbers of the cell type per individual samples, data are presented as mean values ± SEM.bBinary heatmap representing a manually curated list of genes associated with SARS-CoV-2. Orange elements indicate genes with increased expression and white elements indicate genes with decreased expression; Not detected: gene expression was not detected in either of the two tested populations (CLD vs. Control); DEGs with FDR ≤ 0.1 are outlined in black.cDifferential expression analysis for SARS-CoV-2 immune candidate genes in cDCs, Macrophages and Monocytes. *p-adjusted value < 0.1, **p-adjusted value < 0.05,p-adjusted value was Bonferroni adjusted from Seurat FindMarkers differential expression analysis using a negative binomial test and corrected for Age, Ethnicity, Smoking_status and Dataset.dCompared to the healthy control samples, HLA type II score is higher in all disease groups (especially Other-ILD). In the T cell population, cytotoxicity scores (e) and exhaustion scores (f) are higher in the disease samples than in control samples. Ina,d,e, andf: Boxes: interquartile range, lower and upper hinges correspond to the first and third quantiles, upper and lower whisker extends from the hinge to the largest values or smallest values of 1.5 x interquartile range; Tukey_HSD post-hoc test: *pvalue < 0.05, **pvalue < 0.01, ***pvalue < 0.001, ****pvalue < 0.0001. See Supplementary Fig.10for plots with outliers included ford–f. 3c , Supplementary Table 4 ). Among these 20 genes, the tumor suppressor DMBT1 , a glycoprotein that has been shown previously to be highly expressed in ACE2 + AT2 cells [54] and can bind to SARS-CoV-2 spike proteins [55] , and the cartilage acidic protein 1 ( CRTAC1 ), previously known to be downregulated significantly in COVID-19 patients with severe infection [56] , were upregulated in ACE2 + compared to ACE2 - AT2 CLD cells (Fig. 3d ). Next, we sought to identify ACE2 correlated genes in the ACE2 + AT2 cells in different disease groups; thus, identifying the immediate cellular environment SARS-CoV-2 encounters upon infecting a host. We performed Spearman correlation analysis with Benjamini–Hochberg adjusted p values and identified distinct gene profiles significantly correlated with ACE2 for each disease group (Fig. 3c, e ). There were only two ACE2 correlated genes in the Control samples with a cutoff of 99th percentile Spearman rho values and q value less than 0.03, none of those genes are associated with the immune response. In the disease samples, we identified 706 genes (COPD: 330 genes, IPF: 108 genes and Other-ILD: 268 genes) with significant correlation to ACE2 (99th percentile rho values, q value less than 0.03) (Supplementary Dataset 4 ). 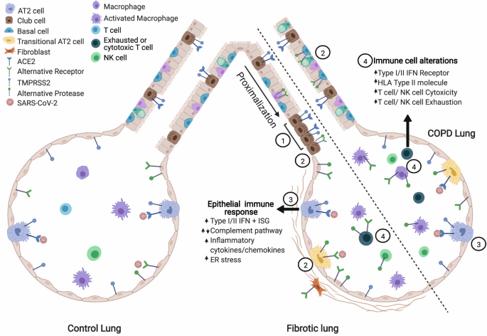Fig. 5: Model of alterations in the diseased lung related to SARS-CoV2 pathogenesis. (1) In the IPF lung, there is a proximalization of the distal airway.ACE2 +epithelial cells cluster in the small airways though totalACE2 +cell numbers are similar to control. (2) The viral entry score (accounting for all described putative receptors and proteases) is increased in diseased lungs. (3) Diseased epithelial cells have alterations in key SARS-CoV-2 response genes/pathways. (4) In the CLD lung, there is increased expression of cytotoxicity and exhaustion genes in immune cell populations and alterations in viral response pathways (interferon, antigen presentation). Figure created in Biorender.com. ACE2 correlated genes are involved in various cellular processes, including viral processes (Supplementary Table 5 ). Many ACE2- correlated genes in the disease samples are associated with the innate and antiviral immune response. In the COPD samples, genes with strong correlation coefficients with ACE2 include several interferon-induced genes ( IFI6, IFIT1, IFIT2 ), a modulator of innate immune function ( OAS1 ), the chemokine receptor ACKR4 , a gene associated with West Nile viral infection ( OASL ), and the ECM regulated transcription factor SOX9 . In the IPF samples, ACE2 expression is strongly correlated with the nuclear factor NXF3 , the transcription factor SP4 , the antiviral factor TRIM11 , and the Forkhead Box Q1 ( FOXQ1 ). In other ILD diseases (non-IPF related), the integrin ITGB8 , a member of the TNF receptor family ( TNFRSF11B ), an important component of the immune response system ( NOD2 ) and an innate immune pathway component ( ITLN1 ) are among the genes with high correlation with ACE2 . The transcription factor FOXQ1 was identified among the 20 unique transcription factors specific for SARS-CoV-2 in a recent in silico study [57] , while OAS1 was among the top 50 genes with a significant correlation coefficient with ACE2 in a previous study [33] . The presence of immune-associated genes in these gene correlation profiles suggests that in patients with CLD, ACE2 + AT2 cells are conditioned and primed to express these genes to cope with viral infection. Baseline differences in inflammatory response programs in chronic lung disease Recent publications have suggested that immune dysregulation, including sustained cytokine production and hyper-inflammation, is associated with SARS-CoV-2 severity [58] , [59] , [60] , [61] . We performed an in-depth examination of the immune cell population to determine whether preexisting immune dysregulation in chronic lung disease patients could contribute to SARS-CoV-2 severity and mortality. We analyzed a total of 421,059 cells from 12 immune cell types (Supplementary Table 3 , Supplementary Fig. 1 ) and found significant increases in the proportion of CD4 T Cells, CD8 T Cells, cDCs and NK cells in the disease groups, most notably in COPD samples (Fig. 4a ). Similar to Fig. 2a , we examined the expression of SARS-CoV-2 and cellular immune response genes in the CLD immune cells. Several genes related to SARS-CoV-2 entry ( CTSL, CTSB, ADAM17) and components of the Interferon and IL6 pathways are significantly dysregulated in the CLD Macrophages and cDCs (Fig. 4b ). Moreover, many immune cells isolated from CLD samples showed elevated levels of genes in the major histocompatibility complex (MHC) class II genes (HLA type II genes) (Fig. 4b ). HLA type II gene module score increased across all disease groups but especially in the Other-ILD samples, compared to controls (Fig. 4d ). Type I IFN response (IFNa score) is slightly elevated in the diseased macrophages and pDCs (Supplementary Fig. 11a ). IL6-associated tocilizumab responsive genes (IL6 score) are expressed at a higher level in the disease groups IPF and Other-ILD, but lower in the COPD samples (Supplementary Fig. 11b ). Previous studies demonstrated elevated exhaustion levels in CD8 T cells in severely affected COVID-19 patients [62] , [63] . All CLD T cells have higher expression levels of cytotoxicity and exhaustion genes compared to controls (Fig. 4e, f ). These perturbations in the T Cell population of CLD lungs may diminish the host immune response to viral infection, leading to a higher risk of severe disease and poor outcomes in response to SARS-CoV-2 infection. Fig. 4: Analysis of SARS-CoV-2 candidate immune response genes in immune cells. a Quantification of cell types as a percent of all immune cells in control and diseased lungs, numbers represent the total numbers of the cell type per individual samples, data are presented as mean values ± SEM. b Binary heatmap representing a manually curated list of genes associated with SARS-CoV-2. Orange elements indicate genes with increased expression and white elements indicate genes with decreased expression; Not detected: gene expression was not detected in either of the two tested populations (CLD vs. Control); DEGs with FDR ≤ 0.1 are outlined in black. c Differential expression analysis for SARS-CoV-2 immune candidate genes in cDCs, Macrophages and Monocytes. * p -adjusted value < 0.1, ** p -adjusted value < 0.05, p -adjusted value was Bonferroni adjusted from Seurat FindMarkers differential expression analysis using a negative binomial test and corrected for Age, Ethnicity, Smoking_status and Dataset. d Compared to the healthy control samples, HLA type II score is higher in all disease groups (especially Other-ILD). In the T cell population, cytotoxicity scores ( e ) and exhaustion scor e s ( f ) are higher in the disease samples than in control samples. In a , d , e , and f : Boxes: interquartile range, lower and upper hinges correspond to the first and third quantiles, upper and lower whisker extends from the hinge to the largest values or smallest values of 1.5 x interquartile range; Tukey_HSD post-hoc test: * p value < 0.05, ** p value < 0.01, *** p value < 0.001, **** p value < 0.0001. See Supplementary Fig. 10 for plots with outliers included for d – f . Full size image To further investigate differences in immune cell type-specific gene expression profiles, we examined expression levels of genes associated with viral infection in disease versus control samples. Amphiregulin (AREG), a ligand for epidermal growth factor receptor, is known to have essential roles in wound repair and inflammation resolution; furthermore, upregulation of AREG is associated with viral infections of the lung [64] . In COVID-19 patients, AREG is significantly upregulated in PBMCs [65] , monocytes, CD4 T Cells, NK cells, neutrophils, and DCs [61] , suggesting that upregulation of AREG may be an attempt to ameliorate the severe injury induced by SARS-CoV-2 infection. We observed reduced expression of AREG in the cDCs and macrophages, but not in the monocytes, in the CLD samples (Fig. 4c , Supplementary Dataset 3 , Supplementary Fig. 12 ). SOCS1 , a suppressor of cytokine signaling, was shown to reduce the type I IFN antiviral response in bronchial epithelial cells after influenza infection [66] , [67] . Expression of the S100A8/A9, members of the S100 family, and the IL6 co-receptor IL6ST was elevated in COVID-19 patients [68] , [69] , [70] . In our study, S100A8/A9 expression is lower in the disease samples in cDCs, macrophages and monocytes while SOCS1 expression is elevated in Other-ILD samples in NK Cells and pDCs (Fig. 4c , Supplementary Dataset 3 ). IL6ST expression level is elevated significantly in COPD and IPF but reduced dramatically in Other-ILD samples in macrophages (log2FC = −2.75, q value = 1.63e-61) (Fig. 4c , Supplementary Dataset 3 ). These basal differences in inflammatory gene expression programs highlight how chronic lung disease alters the inflammatory microenvironment encountered upon viral exposure to the peripheral lung. The COVID-19 pandemic, caused by the SARS-CoV-2 virus, has affected tens of millions of individuals around the globe in just the first nine months of 2020. Patients with CLD have an increased risk for severe SARS-CoV-2 infection: COPD patients have a five-fold increased risk of severe COVID-19 [23] , [24] , [71] , [72] , [73] and ILD patients have up to a four-fold increased odds of death from COVID-19 [28] , [74] . Here, we performed an integrated transcriptomic analysis of scRNA-seq data from healthy and CLD patients to identify potential molecular causative factors determining SARS-CoV-2 severity. To summarize the results (Fig. 5 ): (1) ACE2 and TMPRSS2 are expressed predominantly in epithelial cells and there are no significant differences in the number of ACE2 + cells in all cell types in disease compared to control samples; (2) a viral entry score including multiple entry factors is increased in cells isolated from diseased lungs; (3) CLD epithelial cells, especially AT2 cells, exhibit pre-existing dysregulation of genes involved in viral infection and the immune response; (4) ACE2 protein levels are elevated in the IPF small airway sections; (5) the CLD ACE2 + cells differentially express genes related to SARS-CoV-2 infection compared to CLD ACE2- AT2 cells; (6) a unique ACE2 correlated gene profile for each diagnosis group included antiviral and immune regulatory genes; (7) there are baseline differences in the cellular immune population in disease compared to control samples. Fig. 5: Model of alterations in the diseased lung related to SARS-CoV2 pathogenesis. ( 1 ) In the IPF lung, there is a proximalization of the distal airway. ACE2 + epithelial cells cluster in the small airways though total ACE2 + cell numbers are similar to control. ( 2 ) The viral entry score (accounting for all described putative receptors and proteases) is increased in diseased lungs. ( 3 ) Diseased epithelial cells have alterations in key SARS-CoV-2 response genes/pathways. ( 4 ) In the CLD lung, there is increased expression of cytotoxicity and exhaustion genes in immune cell populations and alterations in viral response pathways (interferon, antigen presentation). Figure created in Biorender.com. Full size image Similar to other coronaviruses, SARS-CoV-2 utilizes cellular receptors ( ACE2 and putatively, BSG, NRP1 and HSPA5 gene products) and priming proteases ( TMPRSS2, CTSL, FURIN ), for viral entry. These factors are expressed predominantly in the upper and lower airways, with ACE2 being expressed highly in nasal goblet and ciliated cells and in a subset of AT2 cells and the absorptive enterocytes in the gut [33] , [34] , [41] , [48] , [51] . We observed a similar expression pattern of ACE2 in our dataset, with AT2 cells having the highest number ACE2 + cells. To our knowledge, publications investigating baseline expression of these SARS-CoV-2 entry factors in lung disease have been limited to asthma and COPD with variable results. For example, studies in asthma patients showed elevated expression of ACE2, TMPRSS2, and FURIN in patients with severe but not mild-moderate asthma [75] , [76] . Leung et al. performed bulk RNAseq and immunohistochemical staining on bronchial epithelial cells and showed significantly elevated expression levels of ACE2 and ACE2 protein in the small airways of COPD patients compared to control [77] . Another study on bronchoscopically isolated tissue showed no relationship between disease status (mild to moderate asthma or COPD) on the expression levels of all SARS-CoV-2 entry factors [42] . Our study utilized scRNAseq technology to study gene expression at a very granular level and did not identify increased ACE2 expression at the single-cell level in CLD, including COPD. However, in the IPF lung, there was a regional concentration of ACE2 + cells in the small airways upon immunohistochemical examination (Fig. 3a, g ), similar to the findings of Leung et al. [77] . While the overall frequency of ACE2 + cells and the ACE2 expression level may be low, changes in the proportional cellular makeup of the diseased lung epithelium may lead to a proportionate increase in ACE2 + “infectable” cells in the distal lung. Importantly, IPF lungs exhibit abnormal expansion of epithelial cell programs, specifically the presence of more proximal specific cell types in the distal lungs [31] , [32] . Thus, our data along with previously published studies together suggest that while overall differences in ACE2 expression and other entry factors may be minimal in CLD, the localization of susceptible cells in the distal lung may promote disease pathogenesis and severity. However, it seems clear that viral entry alone cannot explain the variation in disease severity between patients with and without CLD. In a COVID-19 autopsy study, Dolorey et al . found that in these patients who succumbed to complications of infection, SARS-CoV-2 RNA + cells in the lung were largely in the myeloid lineage and did not overlap with entry factor expression [78] . Thus, once the infection has become established and significant cellular injury has taken place, viral entry factor expression may no longer be essential to continued propagation of injury. A balanced immune response is crucial to viral clearance and avoidance of excessive injury to the host, as evidenced by poor outcomes related both to immunosuppression as well as hyperinflammation in COVID-19 patients [79] . COPD patients with severe COVID-19 had elevated serum levels of various inflammatory cytokines including IL-2R, IL-6, IL-8, IL-10, and TNF-α suggesting there may be global alterations in the immune response [27] . We observed that COPD AT2 cells expressed elevated levels of immune-response related genes ( CSF3, ITGB6, SOCS2 ). G-CSF (encoded by CSF3) is found at high levels in patients with severe COVID-19 and thought to play a role in the hyperinflammatory syndrome while SOCS2 is part of a negative feedback system that regulates the response to cytokines [80] , [81] . ACE2 correlated genes in this cell population were enriched for regulators of the immune response (Fig. 2e ), with several of these genes found to be upregulated in alveolosphere cultures infected with SARS-CoV-2 [36] . In addition to alterations in the cytokine microenvironment, changes in cellular immune populations were also identified in the COPD samples, dysregulation of several genes in inflammatory pathways ( AREG, IL6ST, S100A8/A9, SOCS1 ), and high levels of cytotoxic and exhaustion-related genes in CD4 and CD8 T Cells from COPD lungs. Expression of cytotoxic and exhaustion genes was increased compared to controls but similar in IPF and Other-ILD immune cell types. Together, our data suggest that the immune microenvironment at both the molecular and cellular level in the fibrotic and COPD lung is dysregulated and may promote severe infection and poor outcomes in COVID-19. One limitation of our study is that we focus mainly on the peripheral regions of the lungs, and do not analyze cells in the upper airways or trachea. It is possible that there are significant differences in SARS-CoV-2 entry gene expression between disease and control samples in the more proximal regions of the lungs. Our study is also limited to the expression profiles of patients with CLD without SARS-CoV-2 infection, as samples from patients who are both infected with SARS-CoV-2 and have chronic lung disease are difficult to collect at present. In addition, scRNA-seq is inherently limited to analyses of gene expression which does not always correlate with protein levels. The net effect of many changes in gene expression levels is also difficult to predict and requires determination in experimental models. For example, our analysis demonstrated increased expression of viral entry restriction factors concurrently with an increased viral entry gene score in diseased epithelial cells. Furthermore, scRNA-seq cannot determine spatial relationships which would preclude analysis of cellular behaviors influenced by neighboring cells such as the priming of the viral spike protein by adjacent protease positive cells [82] . Nevertheless, given the inherent limitations in studying human biology, our study highlights crucial areas for future research into the pathogenesis of COVID-19 in patients with CLD including the dysregulation of genes related to viral replication and the innate immune response in epithelial cells, and basal differences in inflammatory cell gene expression programs. scRNA-seq samples scRNA-seq data were obtained from published data with samples in the “VUMC/TGen” dataset from Habermann et al. [32] (GEO accession GSE135893), samples in the “Yale/BWH” dataset came from Adams et al. [31] (GEO accession number GSE136831), samples in the “Pittsburgh” dataset from Morse et al. [30] (GEO accession GSE128033) and samples in the “Northwestern” dataset from Reyfman et al. [29] (GEO accession GSE122960) (Supplementary Tables 1 , 2 ). For specific IRB review of each dataset, please refer to the original paper cited here. In addition, there are 39 unpublished scRNA-seq samples in the “VUMC/TGen” dataset that were collected under Vanderbilt IRB #’s 060165, 171657 and Western IRB # 20181836. scRNA-seq data processing Seurat v4.0 package [83] was used to process the scRNA-seq data. Specifically, for the Pittsburgh, Northwestern datasets and 39 unpublished samples from the VUMC/TGen, the CellRanger (10X Genomics) output files were read into Seurat using the function Read10X , the remaining datasets were already in Seurat format and were loaded using the function readRDS . To eliminate low-quality/dying cells or empty droplets, we removed any cells containing fewer than 1000 genes or more than 25% mitochondrial genes. Due to the large size of the joint dataset, we performed SCTransform [84] for normalization and scaling of each dataset separately, split into four major cell populations using known markers: EPCAM + (Epithelial), PECAM1 + PTPRC - (Endothelial), PTPRC + (Immune) and EPCAM- PECAM- PTPRC- (Mesenchymal). Each population from the four datasets was then merged together to generate four merged Seurat objects (Endothelial, Epithelial, Immune and Mesenchymal). Next, each object was SCTransformed with “dataset” being used as batch_var to eliminate batch effects between datasets. Cell clustering was performed using the Seurat function FindNeighbors and FindClusters and cell type annotation was manually performed on each object using known cell-type specific markers (Supplementary Fig. 1 [32] ). For each cell population, cell type annotation was performed at four levels, ranging from the most general to more granular annotation. Cells expressing more than one cell type specific marker were identified as doublets. After removing doublet cells, all four population datasets were merged to generate the final ILD object containing a total of 611,398 cells and 32 distinct cell types (Supplementary Table 3 , Supplementary Fig. 1 ). Integrated analysis of joint dataset To calculate the percentage of single positive or double positive cells for ACE2 and other cofactors, we counted the number of cells with >0 transcripts of corresponding genes. For double positive, cells have >0 transcripts of both genes of interest. To assess the expression profile of SARS-CoV-2 mediators ( ACE2 , BSG , NRP1, HSPA5) , the corresponding proteases ( TMPRSS2 , CTSL , FURIN ) and other candidate genes involved in SARS-CoV-2 infection in different chronic lung disease subset (COPD, IPF or Other-ILD), we ran the function FindMarkers in Seurat package using the negative binomial test. Using Seurat function CellCycleScoring, we calculated the cell cycle state across all epithelial cells to ensure the cell cycle is not a factor contributing to the differential expression analysis (Supplementary Fig. 7 ). To account for batch effects, we used the parameter “ latent_vars ” to incorporate the four variables (Age, Ethnicity, Smoking status and Dataset) into the negative binomial model. For the binary heatmap, the differential expression analysis was performed between the Disease (including all chronic disease subset) and Control samples. Then, log 2 fold-change was converted into 0 (downregulated in the disease samples) or 1 (upregulated in the disease samples) regardless of the Bonferroni adjusted p values. Heatmaps were generated from the adjusted log 2 FC values using the heatmap.2 function of the gplots R package [85] . For the boxplots, count numbers of selected genes were plotted using the geom_boxplot and geom_jitter function of the ggplot2 R package [86] . Gene module score To calculate the combined expression of genes, we used the AddModuleScore in Seurat v3.1.5 package. SARS-CoV-2 entry gene scores were calculated on SARS-CoV-2 receptors and mediators: ACE2, BSG (CD147), NRP1, HSPA5(GRP78), TMPRSS2, CTSL, FURIN and ADAM17 . Viral entry restriction ISGs: LY6E, CLEC4D, UBD, ELF1, FAM46C, REC8 [43] . Viral replication inhibition ISGs: SPATS2L, ZBP1, DNAJC6, IFIT3, RGS22, IFIT1, IFIT5, B4GALT5 [43] . HLA type II score includes HLA-DRA, HLA-DQA1, HLA-DQA2, HLA-DPA1, HLA-DRB1, HLA-DPB1, HLA-DQB2, HLA-DRB5, HLA-DQB1, HLA-DMA, HLA-DMB . IFN score includes ISG15, IFI44, IFI27, CXCL10, RSAD2, IFIT1, IFI44L, CCL8, XAF1, GBP1, IRF7, CEACAM1 . IL6 scores were calculated on six tocilizumab responsive genes: ARID5A, SOCS3, PIM1, BCL3, BATF, MYC that are associated with the IL-6 pathway [61] . Cytotoxicity associated genes include PRF1, GZMH, IFNG, NKG7, KLRG1, PRF1 [61] and GNLY, GZMB, GZMK [87] . Exhaustion gene set: LAG3, TIGIT, PDCD1, CTLA4, HAVCR2, TOX [63] , and PRDM1, MAF [61] . Significant differences between different groups were calculated using the Tukey_HSD statistic test in the R package rstatix with a confidence level of 0.95 (Supplementary Dataset 2 ). Gene correlation analysis To identify genes that correlate with ACE2 in the AT2 ACE2 + cells, we performed Spearman correlation coefficient analysis on the log-transformed and normalized data using the function cor.test in the R stats v3.6.1 package with Benjamini-Hochberg corrections for p-adjusted values. Gene ontology analysis for the significant correlated genes ( p value ≤ 0.03 and 99th percentile rho) was performed with the Bioconductor R package TopGO version 2.42 and the Bioconductor annotation data package org.Hs.eg.db version 3.12.0; Kolmogorov–Smirnov (KS) statistic method with TopGO default algorithm weight01 test was used for GO term enrichment test [88] , and Benjamini Hochberg (BH) adjusted p values ( q values or FDR) were computed using the R function p .adj. Immunohistochemistry of ACE2 and anti-αvβ6 integrin Formalin-fixed paraffin-embedded histological sections of human lung were cut at 5-microns and dewaxed in xylene prior to rehydration in decreasing concentrations of ethanol. The tissue samples were obtained after informed consent and local ethics approval (South East Scotland SAHSC Bioresource-reference number 06/S1101/41; Brompton Node samples—reference number 15/SC/0101; Papworth Node Samples; non-diseased controls- reference number (Q)GM030404 and Nottingham BRC samples- reference number 08/H0407/1). IHC staining was performed using the Novocastra Novolink™ Polymer Detection Systems kit (Code: RE7280-K, Leica, Biosystems, Newcastle, UK) as previously described [89] . Heat-induced citrate antigen retrieval (pH 6.0) and pepsin antigen retrieval was performed for Rabbit monoclonal ACE2 (ab108252, EPR4435(2) Abcam, UK) and the anti-αvβ6 integrin antibody (6.2A1; Biogen, Cambridge, MA, USA), respectively. Rabbit monoclonal ACE2 (1:400) and anti-αvβ6 integrin (1:3000) was diluted in Leica antibody diluent (RE AR9352, Leica, Biosystems, UK) and incubated with the sections overnight at 4 °C. Novolink DAB substrate buffer plus was used as the chromogen and the slides were counterstained with Novolink haematoxylin for 6 min, dehydrated and cover slipped. A negative control without the application of the primary antibody, and was also used to ensure staining was only related to the presence of the antibody. The immunohistochemically stained slides were scanned using a ScanScope XT Slide Scanner (Leica Aperio Technologies, Vista, CA, USA) under 20× objective magnification (0.5 µm resolution) using Pannoramic Viewer (3DHISTECH Ltd Budapest, Hungary) slide viewing software. Both the percentage of staining and staining intensity of ACE2 expression in lung sections were individually assessed. For ACE2 quantification, the following scoring system of five high-power fields at X40. per tissue section were used: The coding was performed prior to scoring/analysis as: 0 - Negative; 1 - 0–≤10%; 2 - 11–≤25%; 3 - ≤26%. Statistical analyses were completed using GraphPad Prism 7.0 (GraphPad Software, San Diego, CA, USA). One-way analysis of variance was used for comparison of more than two datasets and significant differences between diagnosis groups were calculated using the Tukey HSD test. ACE2 western blot Cell protein was isolated using Cell Lysis Buffer (Cell signalling, USA) supplemented with protease inhibitor cocktail (Sigma, USA) and the quantification performed using BCA Protein Assay Kit (Thermofisher Scientific, UK). Western blotting was performed using 4–12%, pre-cast Bis-Tris gradient gels (Thermofisher Scientific, UK) and 25 µg of protein was loaded per lane. Immunoblots were incubated with anti-ACE2 (ab108252; Rabbit monoclonal-Abcam-EPR4435(2)—1:500 dilution of stock antibody) diluted in 5% skim milk/Tris buffered saline with 0.1% Tween-20 for overnight at 4 °C. A loading control of GAPDH was also used to demonstrate protein loading (ab8245; Mouse monoclonal-anti-GAPDH antibody [6C5] at 1:10000 dilution of stock antibody). Following day immunoblots were incubated with an anti-mouse-HRP and anti-rabbit-HRP conjugated secondary antibodies (Dako, USA) at 1:2500 for 1 hr at room temperature. Visualization was performed with Clarity Max™ ECL Substrate (Biorad, UK) on a Licor C-DiGit. For more information on the anti-ACE2 antibody, please refer to the manufacturer’s datasheet here: https://www.abcam.com/ace2-antibody-epr44352-ab108252.html . Two replicates were performed for the western blot. Statistical analysis Tukey Honest Significant Difference (Tukey_HSD) statistical test from the R package rstatix with a confidence level of 0.95 was used to test statistical dependence of cells expressing the SARS-CoV-2 mediators among chronic disease subsets. Tukey_HSD test was also used to test significant difference in gene expression module score, quantification of cell types and the ACE2 protein expression quantification. Significant differences in gene expression were the Bonferroni adjusted p-values calculated from the FindMarkers function between Control and Disease groups (COPD, IPF, Other ILD) using the fitted negative binomial model and latent_vars parameters as described above. Significance in gene correlation analysis between ACE2 and other SARS-CoV-2 entry factors (Fig. 3a and Supplementary Fig. 10 ) was calculated using Anova. Reporting summary Further information on research design is available in the Nature Research Reporting Summary linked to this article.